Broadly tunable monolithic room-temperature terahertz quantum cascade laser sources Electrically pumped room-temperature semiconductor sources of tunable terahertz radiation in 1–5 THz spectral range are highly desired to enable compact instrumentation for THz sensing and spectroscopy. Quantum cascade lasers with intra-cavity difference-frequency generation are currently the only room-temperature electrically pumped semiconductor sources that can operate in the entire 1–5 THz spectral range. Here we demonstrate that this technology is suitable to implementing monolithic room-temperature terahertz tuners with broadband electrical control of the emission frequency. Experimentally, we demonstrate ridge waveguide devices electrically tunable between 3.44 and 4.02 THz. Mass-producible room-temperature semiconductor sources of tunable coherent terahertz (THz) radiation in the 1–5 THz spectral range are highly desired for sensing, spectroscopy and imaging applications [1] , [2] . Besides p-doped germanium lasers that require strong magnetic fields and low-temperature cryogenic cooling for operation [3] , [4] , quantum cascade lasers (QCLs) are the only electrically pumped semiconductor sources that demonstrated operation in this entire spectral range. Narrowband THz emission has been demonstrated in both THz QCLs [5] , [6] , [7] , [8] and THz sources based on intracavity difference-frequency generation (DFG) in mid-infrared QCLs (THz DFG-QCLs) [9] , [10] . The latter is the only technology that results in electrically pumped monolithic semiconductor sources operable at room temperature in the entire 1–5 THz range [10] , [11] , [12] , [13] . With the introduction of the Cherenkov waveguide scheme [11] , the power output of THz DFG-QCLs has been dramatically improved, with the latest devices producing as much as 215 μW [13] and 1.5 mW [14] peak power output at around 3.5 THz at room temperature. Single-frequency operation with wide continuous tunability is an essential requirement for THz sources for many sensing and spectroscopy applications. The relaxed phase-matching condition of Cherenkov DFG allows one to create THz DFG-QCL tuners with wide tuning range. Spectral tuning of THz DFG-QCLs from 1.7 to 5.25 THz was achieved recently using a diffraction grating in an external cavity setup [12] . However, external cavity tunable laser systems are bulky, have moving parts, and require precise alignment of optical components. Monolithic electrically tunable THz sources would be better suited for many applications owing to their compactness, mass-reducibility potential and intrinsically high reliability due to the lack of mechanical components. The tuning range of monolithic single-mode THz QCLs and THz DFG-QCL sources demonstrated so far is limited to below 30 GHz [15] , [16] , [17] . Efforts to produce tunable THz QCLs by microelectromechanical systems previously resulted in a record 330 GHz tuning around 3.85 THz centre frequency [18] , [19] . Here we report monolithic THz DFG-QCL tuners that can be electrically tuned over 0.58 THz, which is by far the largest tuning range achieved by a monolithic THz tuner to date. Unlike microelectromechanical system-based THz QCLs, our devices operate at room temperature and have no moving parts. Experimentally, our 2.7-mm-long THz DFG-QCL ridge-waveguide device demonstrates electrical tuning from 3.44 to 4.02 THz or over 15% of centre frequency. Design and processing THz tuning in the DFG process ω THz = ω 1 − ω 2 , where ω 1 > ω 2 , can be achieved by changing mid-infrared (mid-IR) pump frequencies, ω 1 or ω 2 . Since a small fractional shift in mid-IR pump frequency translates into a large fractional change of THz emission frequency, this approach leads to monolithic THz semiconductor sources with an extremely wide tuning range. To independently control two mid-IR pump frequencies we create a device with two independently biased distributed grating sections for each pump wavelength. By increasing DC current through these sections, we can electrically tune ω 1 or ω 2 . The mid-IR pump frequencies in our devices can only be red shifted with increase of DC current [20] , [21] , [22] , [23] ; however, THz emission frequency is given by the difference of the two mid-IR frequencies and thus can be both blue and red shifted depending on the choice of the mid-IR frequency to tune. Our proof-of-concept device design is shown in Fig. 1a . It consists of two sections: the front section with a grating designed to select high ( ω 1 ) mid-IR pump frequency and the back section with the grating designed to select low ( ω 2 ) pump frequency. Each section in Fig. 1a can be independently biased and is separated by a gap etched through the heavily doped top waveguide layer to avoid electrical cross-talk (see Methods for a detailed structure of our devices). The top surface grating scheme [21] , [24] , [25] , [26] has been experimentally implemented for frequency selection. The optimal grating etching depth of 170 nm was calculated for our devices, based on the analysis described in ref. 25 . The gratings with such etching depth provide nearly the same coupling constant of ~25 cm −1 for both mid-IR pumps. The grating periods were selected to position the two mid-IR pump wavelengths on both sides of the QCL gain peak as shown in Fig. 1b , which experimentally resulted in the best modal selectivity and the largest single-mode tuning range. The frequency separation between ω 1 and ω 2 was chosen to provide THz emission at 3.5 THz, where the best performance of DFG-QCLs is currently achieved [10] , [11] , [12] , [13] . We fabricated 2.7-mm-long ridge waveguide devices with 22 μm ridge width. The lasers had two 1.2-mm-long grating sections separated by a 300-μm gap. Details of the processing steps are listed in Methods. 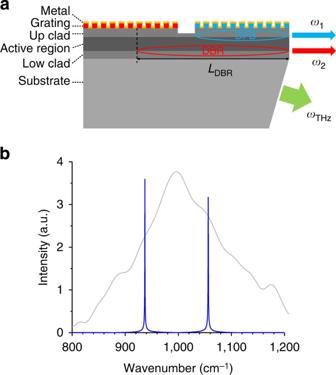Figure 1: Tunable QCL geometry and mid-IR lasing spectra. (a) Schematic of the device, illustrating the front DFB section for the short-wavelength (ω1) mode selection and the back DBR section for the long-wavelength (ω2) mode selection.LDBRindicates the effective cavity length for the DBR laser. Cherenkov THz emission radiates through the polished substrate facet as shown in the figure. (b) Room-temperature emission spectrum (blue) of the 2.7-mm-long device described in the text. The front section of the laser was biased with 1.3 ×Ith(2.4 A) 50 ns current pulses at 50 kHz repetition frequency; the back section of the laser was unbiased. Room-temperature electroluminescence (grey) measured from a circular mesh made of the same QCL material indicates the gain bandwidth of our lasers. Figure 1: Tunable QCL geometry and mid-IR lasing spectra. ( a ) Schematic of the device, illustrating the front DFB section for the short-wavelength ( ω 1 ) mode selection and the back DBR section for the long-wavelength ( ω 2 ) mode selection. L DBR indicates the effective cavity length for the DBR laser. Cherenkov THz emission radiates through the polished substrate facet as shown in the figure. ( b ) Room-temperature emission spectrum (blue) of the 2.7-mm-long device described in the text. The front section of the laser was biased with 1.3 × I th (2.4 A) 50 ns current pulses at 50 kHz repetition frequency; the back section of the laser was unbiased. Room-temperature electroluminescence (grey) measured from a circular mesh made of the same QCL material indicates the gain bandwidth of our lasers. Full size image The lasers were operated by applying pulsed current above a lasing threshold to the front section only. In this configuration the grating in the front section operates as distributed feedback (DFB) grating, while the grating in the back section operates as distributed Bragg reflector (DBR) grating, as shown in Fig. 1a . Wavelength tuning was achieved by applying DC bias below the lasing threshold to either the back grating section or the front grating section. In the latter case the DC bias was supplied through a bias tee. We note that, while temperature tuning is employed to change mid-IR pump frequencies in our proof-of-concept devices, other tuning mechanisms demonstrated in mid-IR QCLs, such as voltage tuning [27] , [28] , [29] , [30] or optical tuning [31] , [32] , [33] , [34] , may be employed as well. Performance Initial device testing was performed by applying pulsed current to the front section only without using any DC bias. Dual-colour single-mode emission with 1/ λ 1 =1,056 cm −1 and 1/ λ 2 =937 cm −1 was observed for pump currents up to 1.6 × I th (1.6 × threshold current), in excellent agreement with the grating design. At pump currents above 1.6 × I th additional lasing modes appeared close to the centre of the gain. The wavelength tuning performance of our devices was investigated at a pulsed pump current of 1.3 × I th applied to the front section, well within the dynamic range of the single-mode pumps operation. Wavelength tuning was achieved by applying DC bias either to the front or to the back section. The tuning rate is expected to be proportional to the temperature change in the laser sections, which is in turn proportional to the dissipated electrical power. 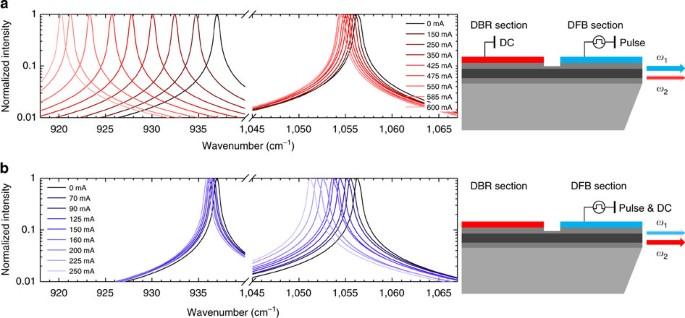Figure 2: Dual-colour mid-IR pump tuning. (a) Right: Device configuration for low-frequency mid-IR pump tuning. Variable DC current (0–600 mA) is applied to the back section; the front section is biased with 1.3 ×Ith(2.4 A) current pulses. Left: Dual-colour emission spectra for different DC bias currents applied to the back section. (b) Right: Device configuration for high-frequency mid-IR pump tuning. The back section is unbiased, while the front section is biased, through a bias tee, with both variable DC current (0–300 mA) and 1.3 ×Ith(2.4 A) current pulses. Left: Dual-colour emission spectra for different DC bias currents applied to the front section. Figure 2 shows the tuning of mid-IR emission spectra as a function of DC current applied to the laser sections. Figure 2a displays the results when the DC bias is applied to the back section of the laser. As expected, the low-frequency pump ω 2 shows significant red shift due to increase in the effective modal refractive index in the DBR section with bias current [20] , [21] , [22] . Figure 2b displays the tuning of mid-IR pumps when DC bias is applied to the front section of the laser. In this case the high frequency ω 1 shows significant red shift. Figure 2: Dual-colour mid-IR pump tuning. ( a ) Right: Device configuration for low-frequency mid-IR pump tuning. Variable DC current (0–600 mA) is applied to the back section; the front section is biased with 1.3 × I th (2.4 A) current pulses. Left: Dual-colour emission spectra for different DC bias currents applied to the back section. ( b ) Right: Device configuration for high-frequency mid-IR pump tuning. The back section is unbiased, while the front section is biased, through a bias tee, with both variable DC current (0–300 mA) and 1.3 × I th (2.4 A) current pulses. Left: Dual-colour emission spectra for different DC bias currents applied to the front section. 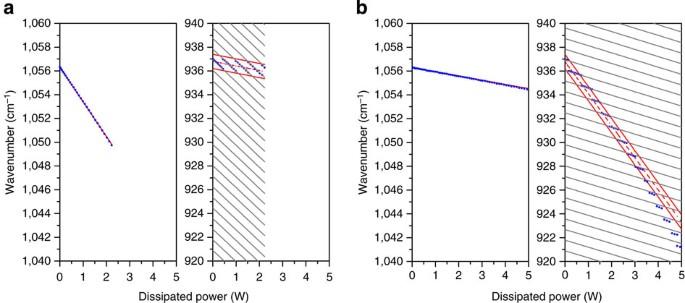Figure 3: Simulated and measured mid-IR tuning behaviour. (a) DC bias on the front DFB section. (b) DC bias on the back DBR section. Blue circles indicate the spectral positions of the measured mid-IR peaks. Red solid lines in both (a) and (b) show the calculated position of the DFB mode (left panels) and the DBR reflection bandwidth (right panels) as a function of dissipated power. Red dashed lines in both left panels indicate the mid-point of the DBR bandwidth. Grey lines in the right panels of (a) and (b) show the calculated laser cavity modes for DBR lasing as a function of DC bias currents. See Methods for details of the computation. Full size image Figure 3 shows more details on the tuning behaviour of the two mid-IR pump frequencies as a function of dissipated DC power, calculated as I DC × V DC , where I DC and V DC are the values of DC current and voltage applied to the laser sections. As expected, the tuning rate is linearly proportional to the dissipated power applied to the tuning section. The spectral position of the high-frequency mid-IR mode ω 1 is determined by the DFB grating in the laser cavity and it changes continuously with temperature. Over 6 cm −1 (0.2 THz) of continuous ω 1 tuning is observed when DC bias is applied to the front section of the laser as shown in Fig. 3a . When the DC bias is applied to the back section of the device, very small tuning of ω 1 is still observed due to heat spreading to the front DFB section of the device (see Fig. 3b ). The evolution of the spectral position of the low-frequency mid-IR mode is more complicated. Principally, it is determined by the position of the laser cavity modes within the high-reflectivity band of the tunable DBR mirror, cf . Fig. 1a . The mid-IR pump ω 2 shows continuous tuning for ~0.5 cm −1 and mode hopping to the next laser cavity mode spaced by ~0.9 cm −1 . This behaviour can be well explained by calculating the effective laser cavity length for the DBR mode of L DBR ≈1.7 mm that gives a mode spacing of 0.88 cm −1 (26 GHz). The calculated dependence of the spectral positions of the DBR laser cavity modes as a function of DBR or DFB bias is shown by the grey lines in Fig. 3 . Details of these calculations are provided in Methods. Over 16 cm −1 (0.4 THz) of ω 2 tuning is achieved when the DC bias is applied to the back section of the device as shown in Fig. 3b . When the bias is applied to the front section, the ω 2 pump mode shows zigzag tuning pattern as the effective laser cavity length changes (see Fig. 3a ). Figure 3: Simulated and measured mid-IR tuning behaviour. ( a ) DC bias on the front DFB section. ( b ) DC bias on the back DBR section. Blue circles indicate the spectral positions of the measured mid-IR peaks. Red solid lines in both ( a ) and ( b ) show the calculated position of the DFB mode (left panels) and the DBR reflection bandwidth (right panels) as a function of dissipated power. Red dashed lines in both left panels indicate the mid-point of the DBR bandwidth. Grey lines in the right panels of ( a ) and ( b ) show the calculated laser cavity modes for DBR lasing as a function of DC bias currents. See Methods for details of the computation. Full size image The spectra of tunable THz emission measured from the laser are shown in Fig. 4a . The linewidth of THz emission was measured to be 10 GHz in the whole tuning range, limited by the spectral resolution of the spectrometer (see Methods). As the DC bias is applied to the back section of the laser, the low frequency of the mid-IR pump ω 2 is red shifted and the frequency separation between the two mid-IR pumps increases, leading to the blue shift of the THz DFG emission. When the DC bias is applied to the front section of the device, the frequency of the mid-IR pump ω 1 is reduced, leading to the red shift of THz DFG emission. A total tuning range of 0.58 THz or over 15% of THz centre frequency is achieved in our devices. Details of the tuning behaviour of THz emission frequency are shown in the lower panel of Fig. 4b . The grey symbols indicate THz emission frequency estimated from the peak spectral positions of the mid-IR pump frequencies shown in Fig. 3 . The red symbols show the measured THz emission frequencies, which are in perfect agreement with expectations. Continuous single-mode tuning near the mode-hope points is achieved by adjusting DC bias voltages to both front and back sections of the laser. Demonstration of continuous tuning across the mode-hope region around 3.6 THz (circled in Fig. 4b ) is shown in the inset of Fig. 4a . To achieve the fine tuning, a second DC bias (DC currents in the range of 0–137 mA) was applied to the DFB section to shift the DFB mode towards the long-wavelength side, while the DBR section was biased at DC currents in the range of 90–170 mA. THz peak power tuning curve is shown in the upper panel of Fig. 4b . For power measurements the device was operated with 1.3 × I th =2.4 A current pulses (50 kHz, 50 ns) applied to the front DFB section. The THz power output is slightly increased at a DFB DC bias power of 500 mW due to the associated increase of the high-frequency ( ω 1 ) mid-IR pump intensity, and then experiences a gradual drop at high DC bias as mid-IR pump powers are reduced. 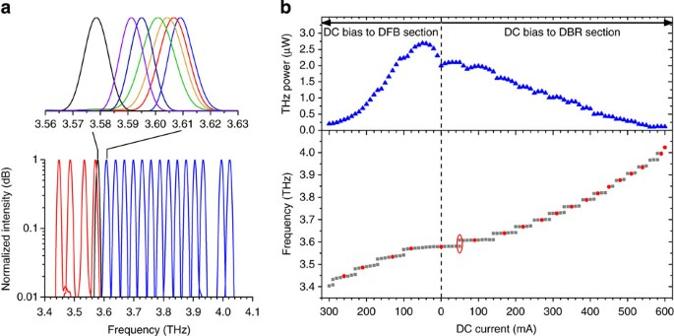Figure 4: THz emission. (a) Electrical tuning of THz emission. Shown are THz spectra for various DC biases applied to the DBR section (blue) or DFB section (red). THz emission spectrum from a device without DC bias applied is shown in black. Top inset: Fine tuning of THz emission around the mode-hop point. (b) Details of THz emission tuning (bottom) and peak THz power (top) of the device as a function of DC current applied to either DFB or DBR section. Grey squares are THz emission frequencies calculated from the frequencies of mid-IR pumps shown inFig. 3. Red circles are experimentally measured positions of THz emission frequencies as shown in (a). The red oval indicates the DBR mode gap filled by the fine tuning shown in (a). For power measurements the device was operated with 2.4 A current pulses (50 kHz, 50 ns) applied to the front DFB section. Figure 4: THz emission. ( a ) Electrical tuning of THz emission. Shown are THz spectra for various DC biases applied to the DBR section (blue) or DFB section (red). THz emission spectrum from a device without DC bias applied is shown in black. Top inset: Fine tuning of THz emission around the mode-hop point. ( b ) Details of THz emission tuning (bottom) and peak THz power (top) of the device as a function of DC current applied to either DFB or DBR section. Grey squares are THz emission frequencies calculated from the frequencies of mid-IR pumps shown in Fig. 3 . Red circles are experimentally measured positions of THz emission frequencies as shown in ( a ). The red oval indicates the DBR mode gap filled by the fine tuning shown in ( a ). For power measurements the device was operated with 2.4 A current pulses (50 kHz, 50 ns) applied to the front DFB section. Full size image Light output–current and current–voltage characteristics of our device measured without any DC bias are shown in Fig. 5a (for mid-IR) and 5b (for THz). Similar to our previous work [12] , [35] , no collection efficiency was introduced to compensate THz power loss through the parabolic mirror setup, which leads to underestimation of THz power. The mid-IR power measurements were performed with an estimated collection efficiency of 100%. Maximum THz peak power was recorded as high as 6.3 μW, with a mid-IR to THz nonlinear conversion efficiency of ~0.4 mWW −2 near the threshold and 0.2 mWW −2 near the rollover point. The reduction of mid-IR to THz conversion efficiency is attributed to reduction of optical nonlinearity due to change in the QCL bandstructure alignment at higher bias voltages as discussed in ref. 12 . 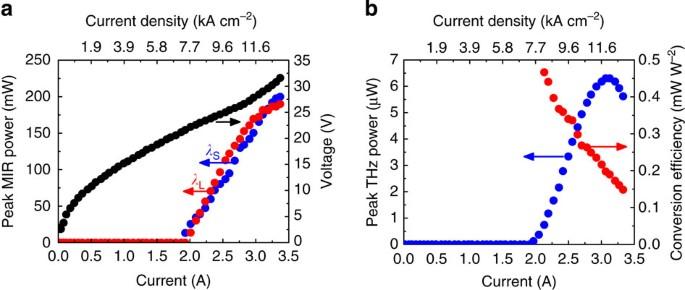Figure 5: Mid-IR and THz peak powers. (a) Light–voltage–current characteristic of the mid-IR pumps. Blue, red and black circles indicate the short-wavelength pump (λS) power, the long-wavelength pump (λL) power and the applied voltage, respectively. (b) Peak THz power and mid-IR-to-THz conversion efficiency. For the measurements shown in (a) and (b) only the 1.2-mm-long and 22-μm-wide DFB section was driven by a pulse current with 50 kHz repetition frequency and 50 ns pulse width at 20 °C. Figure 5: Mid-IR and THz peak powers. ( a ) Light–voltage–current characteristic of the mid-IR pumps. Blue, red and black circles indicate the short-wavelength pump ( λ S ) power, the long-wavelength pump ( λ L ) power and the applied voltage, respectively. ( b ) Peak THz power and mid-IR-to-THz conversion efficiency. For the measurements shown in ( a ) and ( b ) only the 1.2-mm-long and 22-μm-wide DFB section was driven by a pulse current with 50 kHz repetition frequency and 50 ns pulse width at 20 °C. Full size image The tuning range of 580 GHz is, to our knowledge, by far the largest tuning range obtained from a monolithic, electrically pumped single-mode terahertz semiconductor source. We note that we have tested three devices from the same processing batch and all of them demonstrated similar single-mode tuning performance. External cavity tuning of THz DFG-QCL chips [12] and measurements of DFB THz DFG-QCL devices processed from the same wafer [36] indicate that the THz tuning range of monolithic DFG-QCL sources can in principle be extended to span the entire 1–6 THz spectral range and beyond, limited only by the transparency window of InGaAs/AlInAs/InP materials and the rollover of THz DFG efficiency at low THz frequencies [12] , [36] , as long as one finds a way to monolithically tune the mid-IR pump or pumps over a broad spectral range. Recent demonstrations of monolithic single-mode mid-IR QCL tuners based on sampled gratings with over 230 cm −1 (nearly 7 THz) tuning range [37] indicate that future monolithic THz DFG-QCL sources may achieve spectral coverage of the entire 1–6 THz frequency window and beyond. The devices reported here may also be integrated into arrays of lasers, similarly to that demonstrated in mid-IR [38] , to provide continuous spectral coverage over a broad THz spectral range. In conclusion, this work demonstrates that the THz DFG-QCL technology may enable mass production of broadband monolithic semiconductor THz tuners with electrical emission frequency control. As the performance of THz DFG-QCL designs is being improved [12] , [13] , [14] , compact electrically controlled THz DFG-QCL tuners are expected to find applications in a wide variety of THz systems and are expected to dramatically reduce their size and complexity. Device growth and fabrication The laser heterostructure was grown on 350-μm-thick semi-insulated InP substrates using a metal organic vapour phase epitaxy system. A 200-nm-thick InGaAs layer n-doped to 1 × 10 18 cm −3 was grown on top of the substrate for lateral current extraction, followed by a 3.5-μm-thick lower InP cladding layer n-doped to 1.5 × 10 16 cm −3 , a 4.2-μm-thick active region made of two QCL stacks and a 3.5-μm-thick upper InP cladding layer n-doped to 1.5 × 10 16 cm −3 . The growth was finalized with a 500-nm-thick InP outer cladding layer n-doped to 3.5 × 10 18 cm −3 and a 20-nm-thick InGaAs contact layer n-doped to 1 × 10 19 cm −3 . The active-region design was identical to that of the THz DFG-QCL sources reported in ref. 35 . Fixed-frequency THz DFG-QCL processed from this material achieved 40 μW of peak THz power output with 0.36 mWW −2 mid-IR to THz conversion efficiency [35] . We note that the QCL material for our devices was chosen based on material availability and that significantly higher THz power output was reported from Cherenkov THz DFG-QCLs of similar dimensions with more optimal active region and waveguide designs in refs 12 , 13 , 14 . Device fabrication started with removing the InGaAs contact layer and reducing the thickness of the heavily doped InP outer cladding layer from 500 to 100 nm to enhance the coupling between the laser mode and top surface gratings. Rectangular-shaped first-order gratings with 50% duty cycle have been formed using electron-beam lithography. The length of both grating sections is 1.2 mm, resulting in a total cavity length of 2.7 mm, including 300 μm gap between the sections. The 300 μm gap was etched through the remainder of the heavily doped InP outer cladding layer to minimize electrical crosstalk between two sections. The cross-talk resistance between the two grating sections was measured to be 700 Ω at room temperature. This device configuration resulted in the two mid-IR pumps providing roughly equal amounts of optical power near the rollover point. The top DFB/DBR grating period was chosen to be 1.65 μm for the mid-IR pump wavelength of 10.6 μm and 1.48 μm for the mid-IR pump wavelength of 9.5 μm. The gratings were etched to 170±10 nm depth, and 22-μm-wide ridges with grating on top were then processed via dry etching. A 400-nm-thick SiN layer was deposited conformally and opened on top of the ridges for electrical contact. Metal contacts (Ti/Au=20 nm/400 nm) for current injection and lateral extraction were then formed by evaporation and liftoff. Finally, the wafer was cleaved into 2.7-mm-long laser bars and the front facet of the substrate was polished at 30° angle for outcoupling of the Cherenkov radiation [11] . Laser bars were then wire-bonded and mounted on copper blocks using indium paste. Experimental measurements All optical measurements were performed under pulsed bias current with 50 kHz repetition rate and 50 ns pulse width at 20 °C. The mid-IR optical power of each pump was measured using a calibrated thermopile detector. Optical filters were used to perform power measurements for each of the two mid-IR pumps. THz optical power was measured using a calibrated Golay cell detector and off-axis parabolic mirrors under N 2 purged condition to minimize water absorption. Mid-IR and THz spectra were measured using a Fourier-transform infrared spectrometer equipped with a deuterated L-alanine-doped triglycine sulphate detector and a helium-cooled Si bolometer, respectively. The nominal Fourier-transform infrared spectrometer spectral resolution is 0.2 cm −1 for mid-IR and ~0.25 cm −1 for THz measurements. Effective DBR length calculations The cavity mode spacing for the DBR laser is determined by the DBR laser cavity length L DBR , which comprises the length of the front section, the length of the gap and the effective length of the DBR (see Fig. 1a ). The effective DBR length, L eff , corresponds to the effective length of optical power penetration into the grating and is determined by the coupling constant, κ [39] . Assuming the effective refractive index of the DBR section is close to the group index of the Fabry-Perot QCLs, the effective grating length L eff and coupling constant κ can be estimated using the relation [40] , where L g is the physical length of the DBR grating. Taking the value of the coupling constant κ to be 25 cm −1 in accordance with simulations, we obtain L eff as ≈200 μm and total DBR cavity length L DBR as 1.7 mm. The modal spacing for the DBR laser can then be determined as Δ(1/ λ )=1/(2 n g L DBR )≈0.88 cm −1 , where we used n g ≈3.35 (refs 11 , 41 ). This result is in excellent agreement with the experimental measurement of 0.9 cm −1 . 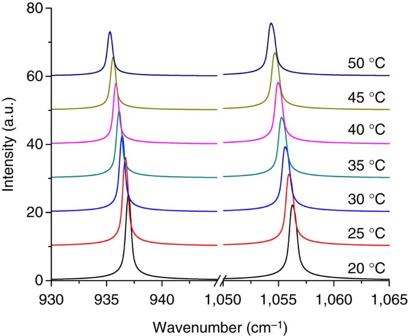Figure 6: Temperature dependence of Mid-IR spectra. Mid-IR emission spectra at various heat sink temperatures of the device operated in pulsed mode without DC bias current. Temperature increase in the laser sections Figure 6 shows the emission frequency of the device discussed here as a function of heat sink temperature. The laser was operated with 50 ns pulsed current and no DC bias was applied to any of the laser sections. The data in the figure allow us to estimate the temperature tuning rate d(1/ λ )/d T in our device to be −0.064 cm −1 K −1 for the high mid-IR pump frequency ( ω 1 ) and −0.056 cm −1 K −1 for the low mid-IR pump frequency ( ω 2 ). We can then use these coefficients to deduce the temperature change in the DFB and DBR sections of our device for the different applied DC powers shown in Fig. 3 . We obtain the maximum bias-induced temperature increase in the DFB and DBR sections as ~100 and 250 °C, respectively. Figure 6: Temperature dependence of Mid-IR spectra. Mid-IR emission spectra at various heat sink temperatures of the device operated in pulsed mode without DC bias current. Full size image Heat diffusion between the DFB and DBR sections Figure 3 shows the dependences of the mid-IR emission frequencies in our device on the DC power applied either to the DFB section or to the DBR section. Nearly linear dependence of the frequency change on the applied DC power is observed in all cases. In particular, the tuning rate of the DFB mode was measured to be −2.94 cm −1 W −1 when the DC bias was applied to the DFB section and to be −0.37 cm −1 W −1 when the DC bias was applied to the DBR section. Given the above values of d(1/ λ )/d T coefficients, we obtain the average temperature increase rates in the DFB section as 45.9 and 5.8 K W −1 when the DC power is applied to the DFB section and the DBR section, respectively. Since the device has symmetric geometry, the same picture applies for temperature increase in the DBR section. Laser tuning characteristics The spectral position of the DFB lasing mode is determined by the Bragg wavelength of the DFB grating and one expects continuous tuning of the DFB lasing mode as DFB section temperature continuously changes, assuming the mirror reflectivity is negligible. In contrast, the spectral position of the DBR mode is determined by the position of the laser cavity mode closest to the DBR mirror reflectivity peak, and mode-hopping behaviour of the DBR laser emission is expected as DBR section temperature changes. The relative shift of the spectral position of the DFB mode is given as where n eff_DFB (Δ n eff_DFB ) is the value (change in value) of the effective refractive index of the laser mode in the DFB section. The relative frequency shift of the peak of DBR mirror reflectivity (Δ v B-DBR / v B-DBR ) and the frequency change in the cavity mode position (Δ v C / v C ) as a function of the change of refractive indices in different sections of our device can be expressed as [40] , where n eff_DBR (Δ n eff_DBR ), n eff_gap (Δ n eff_gap ), and n eff_DFB (Δ n eff_DFB ) are the values (change in values) of the effective refractive indices of the long-wavelength laser mode ω 2 in the DBR section, in the gap between the DBR and DFB sections, and in the DFB section, respectively, L DFB is the length of the DFB section, L gap is the length of the gap between DFB and DBR sections and L eff is the effective grating length for the DBR section defined earlier. In our analysis we have assumed n eff_DBR ≈ n eff_gap ≈ n eff_DFB for simplicity. As DC bias on the DFB section increases, the effective refractive indices in different sections of our device increase due to temperature rise. The process can approximately be expressed as where is the dissipated power applied to the DFB section, and , and are the effective refractive index tuning coefficients in the DFB, DBR and gap sections, respectively. The values of and are determined from the experimental data on modal tuning shown in Fig. 3a , using the relation, , where Λ is the grating period and λ is the emission wavelength. Equations (3), (5) and (6) were used to plot the positions of the DBR laser cavity modes in the right panel in Fig. 3a . The contribution of Δ n eff_gap was ignored in the simulation due to its relatively short length though it can also be used as a fitting parameter. Similarly, as DC bias on the DBR section increases, the effective refractive indices in various sections of the device change according to the expressions: where is the dissipated power to the DBR section; , and are the effective refractive index tuning coefficients in the DBR, DFB, and the gap sections, respectively. The values of and are obtained from the experimental data on modal tuning shown in Fig. 3b as described above. Equations (3), (7) and (8) are then used to plot the position of the DBR laser cavity modes in the right panel in Fig. 3b . The contribution of Δ n eff_gap was ignored in the simulation for the same reason noted above. How to cite this article: Jung, S. et al . Broadly tunable monolithic room-temperature terahertz quantum cascade laser sources. Nat. Commun. 5:4267 doi: 10.1038/ncomms5267 (2014).